Magnetoelectric quasi-(0-3) nanocomposite heterostructures Magnetoelectric composite thin films hold substantial promise for applications in novel multifunctional devices. However, there are presently shortcomings for both the extensively studied bilayer epitaxial (2-2) and vertically architectured nanocomposite (1-3) film systems, restricting their applications. Here we design a novel growth strategy to fabricate an architectured nanocomposite heterostructure with magnetic quasiparticles (0) embedded in a ferroelectric film matrix (3) by alternately growing (2-2) and (1-3) layers within the film. The new heteroepitaxial films not only overcome the clamping effect from substrate, but also significantly suppress the leakage current paths through the ferromagnetic phase. We demonstrate, by focusing on switching characteristics of the piezoresponse, that the heterostructure shows magnetic field dependence of piezoelectricity due to the improved coupling enabled by good connectivity amongst the piezoelectric and magnetostrictive phases. This new architectured magnetoelectric heterostructures may open a new avenue for applications of magnetoelectric films in micro-devices. With the development of new devices miniaturizing technology, there is growing interest in combining electronic and magnetic properties into multifunctional thin-film materials for potential applications in novel devices [1] , [2] , [3] , [4] . Magnetoelectric (ME) materials, which would exhibit an induced polarization/magnetization under external magnetic field/electric field, are especially attractive because they not only bear the properties of individual polar and spin subsystems but also exhibit additional product functionalities due to the ME interactions between them [5] , [6] , [7] , [8] . Compared with single-phase ME materials, ME composites of piezoelectric and magnetostrictive components are particularly appealing due to their much higher ME coefficients and maximum operational temperatures [9] , [10] . For such composites, the ME effect is a product property of the piezoelectric and piezomagnetic coefficient of the corresponding phases [11] . The average ME properties can be tailored by choosing not only suitable individual component phases but also composite architectures. On the micro- or nano-scale, the current phase connectivity architectures, which have been extensively studied for the ME composite thin films, can be summarized by two types: (i) vertical heteroepitaxial nanocomposites with nanorods of one phase embedded in a matrix of the other (named as 1-3) (refs 12 , 13 , 14 , 15 , 16 ); and (ii) multilayering (named as 2-2) (refs 17 , 18 , 19 , 20 , 21 ). However, there are shortcomings for both of these forms: the effective ME coupling of the (2-2) film connectivity is limited by the clamping of films to the substrate [22] , while the low resistivity of the interconnected ferromagnetic phase of the (1-3) structure lowers the net resistivity of the composite layer, which in turn provides a path for dielectric leakage current. Here we propose a new concept to overcome the limitation of both the (2-2) and (1-3) phase connectivities by alternately growing (2-2) and (1-3) layers within the film, and demonstrate the formation of a new quasi-(0-3) heterostructure with magnetic quasiparticles (0) embedded in a ferroelectric film matrix (3). Different from the previously reported (0-3) composites [23] , [24] , [25] with a randomly distributed magnetic phase component embedded in a matrix, the designed new structure has a somewhat orderly arranged magnetic nanorod particles with the same height and approximate similar planar area as those of the middle layer. Such a new structure overcomes the clamping effect from the substrate of the (2-2) connectivity, while significantly reducing the leakage current paths through the ferromagnetic phase of the (1-3) structure. As a result, the connectivity amongst the constituent phases shows an improved ME coupling along the vertical direction due to the improved physical and electrical contact between piezoelectric and magnetostrictive phases on all sides, enhancing thereby the potential for ME effects. This opens up a new avenue of approach for the ME heterostructures in micro-device applications. Preparation and characterization of the heterostructures Films were grown on (001) oriented SrTiO 3 (STO) substrates using pulsed laser deposition by alternately using targets of pure BiFeO 3 and of a 65:35 BiFeO 3 -CoFe 2 O 4 (BFO-CFO) solid solution. 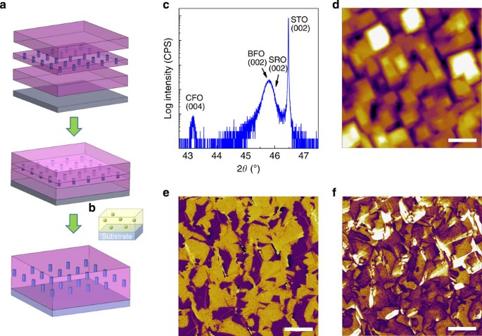Figure 1: Film growth process and structural characterization. (a,b) Sketch of the film growth process for nanocomposites of CFO spinel pillars inside a BFO perovskite matrix (a) and of the heterostructure similar to the (0-3) particulate composite (b). (c)2θ-ωX-ray scans for the film. (d–f) AFM topography (d) PFM out-of-plane phase (e) and amplitude (f) images of the film. Scale bar, 1 μm. Figure 1a shows the film growth process and a schematic diagram of the as-grown quasi-(0-3) heterostructures, which comprise of CFO magnetic nanorod particles embedded in a BFO ferroelectric film matrix. X-ray diffraction reveals that the nanostructure is highly orientated on the substrate. Further 2 θ-ω scans show a relationship of BFO (002) // STO (002) between the perovskite BFO phase in the matrix of the film and the STO substrate ( Fig. 1c ). A (002) SrRuO 3 (SRO) layer, which is used as a bottom electrode for property measurements, is also closely oriented to the BFO (002). A single crystal (004) peak for the spinel CFO nanorod particles in the film is also clearly identified. Figure 1d shows an atomic force microscopy (AFM) image of the surface morphology, from which a uniform square BFO grain array is identified on the surface. The corresponding piezoresponse force microscopy (PFM) images reveal good piezoelectric properties ( Fig. 1e,f ). The domain structures are not constrained by grain boundaries, revealing good low-angle boundaries between grains. This type of semi-coherent grain boundary will benefit strain transfer between phases in the nanocomposite. Figure 1: Film growth process and structural characterization. ( a , b ) Sketch of the film growth process for nanocomposites of CFO spinel pillars inside a BFO perovskite matrix ( a ) and of the heterostructure similar to the (0-3) particulate composite ( b ). ( c ) 2θ-ω X-ray scans for the film. ( d – f ) AFM topography ( d ) PFM out-of-plane phase ( e ) and amplitude ( f ) images of the film. Scale bar, 1 μm. Full size image To reveal microstructures of the films, we conducted cross-sectional transmission electron microscopy (TEM) imaging, as shown in Fig. 2 . The CFO phase (indicated by arrows in Fig. 2a ) is found to be embedded in the BFO matrix phase in the middle of the original BFO–CFO layer in a somewhat ordered fashion and the BFO bottom and top layers are well connected through the BFO matrix, forming a three-layer quasi-(0-3) heterostructure. With a size of about 500 nm lateral and 300 nm vertical, these particles are a little large to be deemed as (0) for those CFO particles. However, with regard to the film size and considering the surrounding matrix that the particles are embedded, it seems appropriate to refer to this composite phase connectivity as a ‘quasi-(0-3) structure’. In 2013, Stratulat et al . [26] reported a novel method about self-assembly process, which was based on patterning the nucleation points through a hard mask, to create large areas of perfectly ordered film with first phase pillars embed in second phase matrix. Similar to this novel process, we also obtained orderly distributed ferromagnetic phase inside ferroelectric matrix by simple method. Energy-dispersive X-ray spectroscopy (EDS) mapping identifies chemically the individual (well-aligned) nanorod particles as CFO, as the Bi concentration is low, while the Co concentration is high ( Fig. 2b ). In addition, no signals from any impurity elements in the film are identified in the EDS spectrum, indicating that no significant amounts of impurities are introduced during sample preparation. Analysis of selected-area electron diffraction patterns shows that the nanorod particles are of single phase with [112] zone axis ( Supplementary Fig. 1 ). Furthermore, the selected-area electron diffraction patterns taken from a region larger than a nanorod particle reveal two sets of reflections, which belong to the BFO and CFO phases, indicating that no additional third phases form in the layer. To extract atomic-scale information, we present atomic-resolution high-angle annular dark-field (HAADF) scanning TEM (STEM) images ( Fig. 2d,e ). Since the intensity of an atomic column is approximately proportional to Z 1.7 ( Z : atomic number), brighter spots on the BFO side represent Bi columns, while darker ones represent Fe ones; whereas on the CFO side, brighter spots are Fe columns that have a double concentration relative to other Fe columns that are darker, and the other darker columns are Co and O columns. In addition, one can notice that the interface is near atomically abrupt and coherent with no amorphous layers, secondary-phase layers, contaminants or transition regions. This confirms a clean and direct contact of CFO to BFO at the atomic scale ( Fig. 2d ). The CFO nanorod particles maintain the spinel structure without clear evidence of inter-diffusion, even though they are embedded in the BFO matrix. These findings are also corroborated by annular bright-field (ABF) STEM images, where the O atomic columns can also be identified ( Supplementary Fig. 2 ). 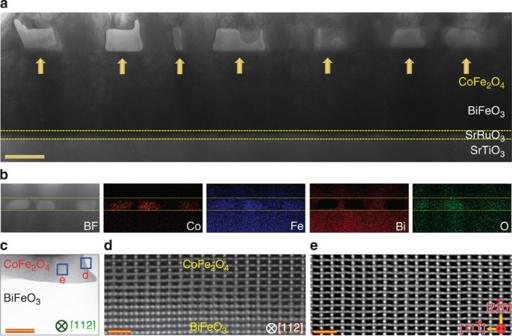Figure 2: Structural and chemical analysis of the nanocomposite films. (a) A TEM image of the nanocomposite film. The CoFe2O4phase is indicated by arrows. Scale bar, 500 nm. (b) A TEM image of the film and corresponding energy-dispersive X-ray spectroscopy (EDS) mapping of the Co, Fe, Bi and O. (c) Aberration-corrected STEM image of the interfaces in the nanocomposite films viewed from [112] direction. Scale bar, 200 nm. (d,e) Atomic-resolution HAADF STEM images at the CFO/BFO interface (d) and within the CFO film (e). Scale bar, 1 nm. The locations of the images are highlighted inc. Figure 2: Structural and chemical analysis of the nanocomposite films. ( a ) A TEM image of the nanocomposite film. The CoFe 2 O 4 phase is indicated by arrows. Scale bar, 500 nm. ( b ) A TEM image of the film and corresponding energy-dispersive X-ray spectroscopy (EDS) mapping of the Co, Fe, Bi and O. ( c ) Aberration-corrected STEM image of the interfaces in the nanocomposite films viewed from [112] direction. Scale bar, 200 nm. ( d , e ) Atomic-resolution HAADF STEM images at the CFO/BFO interface ( d ) and within the CFO film ( e ). Scale bar, 1 nm. The locations of the images are highlighted in c . Full size image Ferroelectric and ferromagnetic properties Ferroelectric ( P – E ) hysteresis measurements ( Fig. 3a ) at room temperature reveal the ferroelectric nature for the BFO phase of the heterostructures. The saturation polarization is P s =77 μC cm −2 , with a remnant polarization of P r =68 μC cm −2 and a coercive field of E c =33 kV mm −1 . The P – E loops are slightly asymmetric, implying that an internal bias field exists at the interface between electrode and thin film, that is, the loops can be saturated in forward and reverse directions. These values are considerably higher compared with prior studies of the P – E loops for (1-3) BFO–CFO films, which have values of P s =53 μC cm −2 , P r =34 μC cm −2 and E c =20 kV mm −1 . Clearly, the ferroelectric properties are altered by the quasi-(0-3) connectivity obtained by pre-depositing and post-depositing bottom and top BFO layers. The heterostructured film has a higher resistivity than the two-phase BFO–CFO middle layer, which enables retention of charge and allows better measurement of the dielectric displacement current of the polarization. 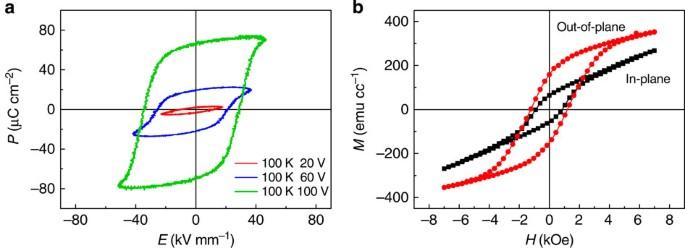Figure 3: Ferroelectric and magnetic properties of nanocomposite films. (a)P–Ehysteresis loops for the quasi-(0-3) BFO/BFO–CFO/BFO nanocomposite film. (b)M–Hhysteresis loops along the in-plane and out-of plane directions for the quasi-(0-3) BFO/BFO–CFO/BFO nanocomposite film. The magnetization is normalized to the volume fraction of the CFO phase. Figure 3b shows magnetic M – H hysteresis loops of the BFO/BFO–CFO/BFO quasi-(0-3) heterostructures using both in-plane and out-of-plane measurement configurations. The magnetization values are normalized to the volume fraction of the CFO phase in the film. Although the shapes of M – H loops for the in-plane and out-of-plane directions are found to be similar to those previously reported for single phase CFO and (1-3) self-assembled BFO–CFO films [27] , [28] , [29] with nearly equal coercive field H c values, the remnant magnetization M r along the in-plane direction is lower than that along the out-of-plane direction. For the quasi-(0-3) heterostructures, the CFO nanorod particles in the template layer are dimensionally isolated [30] . So the spin state is less stable along the in-plane direction than the out-of-plane one, which makes spin rotation easier. It has been shown that the epitaxial CFO films grown on STO are compressed along in-plane direction. Since CFO has a considerable negative magnetostriction, the magnetoelastic energy makes a notable contribution to the total energy, which in turn forces the out-of-plane direction to be the easy axis. Small residual strain in the BFO-CFO layers may cause the existing of anisotropy between the in-plane and out-of-plane directions. Note that the top and bottom BFO layers maintain the strain state of the middle BFO–CFO layers, imposing insignificant effects on its magnetic properties. Figure 3: Ferroelectric and magnetic properties of nanocomposite films. ( a ) P – E hysteresis loops for the quasi-(0-3) BFO/BFO–CFO/BFO nanocomposite film. ( b ) M – H hysteresis loops along the in-plane and out-of plane directions for the quasi-(0-3) BFO/BFO–CFO/BFO nanocomposite film. The magnetization is normalized to the volume fraction of the CFO phase. Full size image Magnetic field dependence of piezoelectricity The new heterostructure may also possess good piezoelectricity and ME properties. PFM switching characteristic measurement before and after applying a controllable d.c. magnetic bias confirms the presence of piezoelectricity and ME coupling in the BFO/BFO–CFO/BFO quasi-(0-3) heterostructures [7] . A sequence of triangle square d.c. voltages pulses [31] accompanied with a.c. voltage are used to the sample through the conductive tip for achieving the switch of the polarization of the BFO phase in the heterostructure. Meanwhile, the corresponding piezoresponse is also measured. Fig. 4a and b show PFM amplitude and phase signal, which are the generated characteristic butterfly loops and hysteresis loops, respectively. The amplitude and phase are measured using a pulse-on-and-off triangle–square waveform. The advantage for the signal obtained while the pulse is off is that the electrostatic effect is pronouncedly reduced [32] . The average phase contrast curves of switching with the d.c. magnetic bias and without the bias are shown in Fig. 4b , which are found to be close to 180°, consistent with the phase changed from the polarization switch [33] . The maximum displacement (PFM amplitude) is 43 p.m. without external magnetic bias with about 9 V of the corresponding coercive voltage. In comparison, under a 2900 Oe external magnetic bias, the maximum displacement is increased to 51 p.m. with the enhancement of the corresponding coercive voltage to 12 V. This demonstrates that electrical properties are changed by the applied magnetic field, indicative of a ME coupling in the heterostructure. 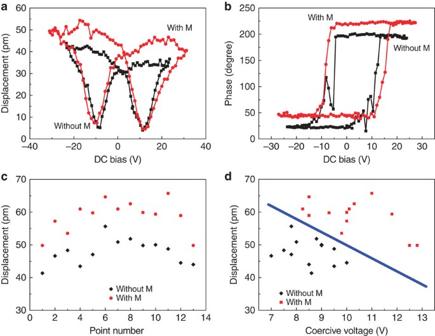Figure 4: Piezoelectric properties and indirect ME effect of nanocomposite films. (a,b) The switching characteristics of piezoresponse for quasi-(0-3) BFO/BFO–CFO/BFO nanocomposite film with and without the application of external magnetic field: the displacement-voltage butterfly loop (a) and the phase-voltage hysteresis loop (b). (c,d) Statistical chart for the piezoresponse displacement value difference with and without the application of external magnetic. The measured piezoresponse displacement as a function of each selected area (c) and the coercive field (d) in the same measurement area. The external magnetic is adopted to be 2,900 Oe. Figure 4: Piezoelectric properties and indirect ME effect of nanocomposite films. ( a , b ) The switching characteristics of piezoresponse for quasi-(0-3) BFO/BFO–CFO/BFO nanocomposite film with and without the application of external magnetic field: the displacement-voltage butterfly loop ( a ) and the phase-voltage hysteresis loop ( b ). ( c , d ) Statistical chart for the piezoresponse displacement value difference with and without the application of external magnetic. The measured piezoresponse displacement as a function of each selected area ( c ) and the coercive field ( d ) in the same measurement area. The external magnetic is adopted to be 2,900 Oe. Full size image To confirm the presence of a ME effect, we conducted multiple measurements from many areas of the films. A statistics chart ( Fig. 4c ) is made for the piezoresponse displacement value difference, which is measured at the same points before and after the application of external magnetic bias for the various sample areas. The measured piezoresponse displacement value under magnetic field (~58.7 p.m. on average) is larger than that without magnetic field (~47.9 p.m. on average). The confidence interval for both piezoresponse displacement before/after applied magnetic field are shown on Supplementary Table 1 . Moreover, since a slight increase in the coercive field E c is observed after the application of external magnetic bias, we provide another statistical chart ( Fig. 4d ) summarizing the piezoresponse displacement and the difference in the E c value for the measurement points before and after application of external magnetic bias for comparison. One can clearly see that the data fall in two groups: the black points with a relatively smaller piezoresponse displacement and E c values before applying the magnetic bias, and the red ones with an enhanced piezoresponse displacement and E c after applying magnetic bias (separated by a blue line). These results confirm the ME effect in the new quasi-(0-3) heterostructures. The switching characteristics of the piezoresponse of the heterostructures from various sample regions (with the statistics given) show changes in electric polarization upon applying magnetic bias. On the basis of piezoresponse displacement values changing with the absence/presence of magnetic field, combined with the statistics method, the lateral ME coefficient α 31 for the quasi-(0-3) heterostructures was calculated by following Xie's approach [7] ( Fig. 4a ). Here, the application of a lateral magnetic field of ▵ H 1 =2,900 Oe has induced the longitudinal electric field change ▵ E 3 , and the lateral ME coefficient is α 31 = ▵ E 3 / ▵ H 1 . From the average change in the displacement ▵ u with and without magnetic field, the electric field change can be obtained as ▵ E 3 = ▵ u / d 33 D . From the displacement-voltage loop, without the magnetic field, we could calculated the piezoelectric coefficient d 33 by d 33 = u / V . And V is the applied a.c. voltage (using 1V here) which used to induce piezoelectric vibration in our experiment. By taking a mean ▵ u value of 10.8 p.m. and a mean u of 47.9 p.m., which are both measured in a remnant state when the d.c. voltage equals zero in the displacement-voltage loops, with the measured film thickness D of about 2.3μm, the ▵ E 3 is calculated to be 9.8 × 10 5 mV cm −1 , giving rise to α 31 =338 mV cm −1 Oe −1 . This value is several times higher than those of the (0-3) type composite films reported previously [25] , [34] , indicating enhanced atomic-scale tight binding between the two constituting phases during the film growth process. The unique heterostructure of the films can account for the observed property shifts. The changes in the BFO piezoresponse with magnetic bias applied across the CFO nanopillars demonstrate a strain-mediated ME coupling between magnetostrictive and piezoelectric phases in the intermediate BFO–CFO layer. Upon applying an in-plane magnetic field, the CFO nanopillars undergo a remarkable in-plane contraction and out-of-plane elongation due to the large negative magnetostriction constant λ 100 of −590 p.p.m. (ref. 35 ). Given the good lattice coherency between the CFO nanopillar and BFO matrix ( Fig. 2d,e ), the in-plane compressive magnetostrictive strains can be effectively transferred to the BFO regions at close to the top and bottom surfaces of the CFO pillar, which in turn expands the out-of-plane lattice parameters of the BFO therein. On the other hand, the out-of-plane tensile magnetostrictive strains can directly stretch the BFO regions along the lateral surfaces of the CFO. Both processes stabilize the polarization along the out-of-plane <111> axes, which therefore accounts for the increase in the E c ( Fig. 4b ). These magnetostrictive strains transferred from the CFO also account for the increase in the piezoresponse ( Fig. 4a,c,d ). For clearer illustration, we performed phase-field simulation (see the model setup in Fig. 5a and details in Methods) for the present quasi-(0-3) nanocomposite heterostructure. 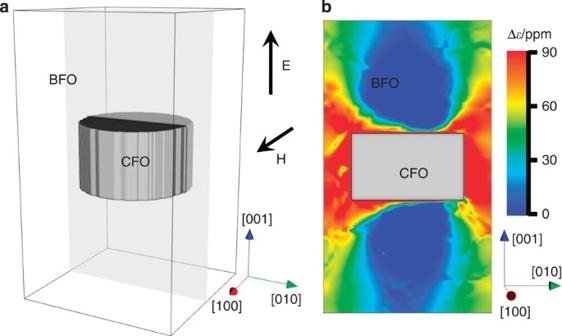Figure 5: Phase-field simulation on the piezoelectric response of the nanocomposite film. (a) Schematics of the phase-field model. (b) Distribution of the out-of-plane piezoelectric strain response enhancement Δεin the cross-section plane (as shown by the grey translucent plane ina) to an electric voltageU=20 V, after application of an external magnetic field along the in-plane [100] direction. Figure 5b shows the simulated enhancement of the piezoelectric strain. The BFO regions along the lateral surfaces of the in-plane-magnetized CFO pillars are subjected to the out-of-plane tensile magnetostrictive strains and gains polarizability along the out-of-plane direction, making primary contribution to the piezoresponse enhancement. On the other hand, although the BFO regions adjacent to the top and bottom surfaces of the CFO nanopillar also exhibit an appreciable enhancement in the out-of-plane piezoelectric strain response, the magnitude of enhancement is much smaller because of the smaller contacted surface area. Our simulation results also suggest an increase of 23.6% in the average out-of-plane piezoelectric strain from 165 to 204 p.p.m. on the application of in-plane magnetic field, consistent with the experimentally observed 22.5% increase in the out-of-plane piezoelectric displacement ( Fig. 4a ). Figure 5: Phase-field simulation on the piezoelectric response of the nanocomposite film. ( a ) Schematics of the phase-field model. ( b ) Distribution of the out-of-plane piezoelectric strain response enhancement Δ ε in the cross-section plane (as shown by the grey translucent plane in a ) to an electric voltage U =20 V, after application of an external magnetic field along the in-plane [100] direction. Full size image Achieving a better coupling between the piezoelectric and magnetostrictive components is a key point to obtain an enhanced ME effect in the ME composites. We have developed a novel growth strategy and fabricated a new architectured nanocomposite heterostructure by combining the structural advantages of the (2-2) and (1-3) phase connectivity. The phase distribution in the heteroepitaxial films not only overcomes the clamping effect from substrate (inherent to (2-2) connectivity) but also significantly reduces the leakage current paths through the ferromagnetic phase (inherent to (1-3) connectivity). We also identify an indirect ME effect by the switching characteristics of the piezoresponse for the heterostructure, and demonstrate that the improved connectivity amongst the constituent phases results in a better coupling between the piezoelectric and magnetostrictive phases, yielding notable ME effects. Such new quasi-(0-3) ME heterostructures and their combination of properties hold substantial promise for multifunctional micro-device applications. Sample growth An epitaxial BiFeO 3 bottom layer thin film was first grown on (001) oriented STO substrates by pulsed laser deposition. Two-phase 0.65BiFeO 3 –0.35CoFe 2 O 4 thin films were thereafter deposited on top of BFO film as a middle layer. This self-assembled layer was then used as a template, onto which a third BiFeO 3 top layer was deposited. All three layers were deposited at 700 °C under a 90 mTorr oxygen partial pressure. The films were deposited using a Lambda 305i KrF laser with a wavelength of 248 nm, focused to a spot size of 2 mm 2 , and incident on the surface of a target at an energy density of 3 J cm −2 . The distance between the substrate and target was 6 cm and the base vacuum of the chamber was 10 −5 Torr. Structure characterization The crystal structures of thin films were determined using a Philips X’pert high resolution X-ray diffractometer equipped with a two-bounce hybrid monochromator and an open three-circle Eulerian cradle. The surface topology and piezoresponse of the BFO–CFO thin films were studied with MFP-3D atomic force microscopy (Asylum Research, Santa Barbara, CA). The PFM studies were carried out on DART (dual AC resonance tracking) mode [36] with a drive amplitude (AC voltage) of 1.5 V applied to the tip. The used conductive cantilever was Asylmelectric (Ti/Ir coating) with a resonance frequency of around 70 kHz and a spring constant of 2 nN nm −1 . The contact resonant frequency in the DART mode was around 280 kHz. Cross-section thin-foil specimens for TEM and STEM observations were prepared by cutting, grinding and dimpling the samples down to ~20 μm. In the Ar ion-beam thinning process, we applied a gun voltage of 1–4 kV and an incident beam angle of 4–6° to avoid radiation damage. SADP, EDS and TEM images were taken using a JEOL JEM-2010F operated at 200 kV. HAADF and ABF images were observed using a 200-kV ARM-200FC STEM equipped with a probe corrector (CEOS GmbH), providing an unprecedented opportunity to probe structures with sub-Ångström resolution. For the HAADF imaging, a probe convergence angle of ~22 mrad and a detector with an inner semiangle of over 60 mrad were adopted. The ABF STEM images were taken using a detector of 6–25 mrad. Electrical and magnetic measurements Ferroelectric P – E hysteresis loops were measured by a modified Sawyer-Tower circuit. Magnetic hysteresis loops were measured using a vibrating sample magnetometer (VSM 7304, Lake Shore Cryotronics, Westerville, OH). The coupling of electric and magnetic measurements were done on a MFP-3D (Asylum Research) AFM equipped with one external varied field magnet (VFM, Asylum Research). The sample was placed on the VFM module that was compatible to the AFM scanner. For the point piezoresponse measurement, a triangle–square waveform with the amplitude of 30 V was applied to the tip, accompanying with 1 V AC bias. After the switching curve was achieved, the in-plane magnetic field was increased to 2,900 Oe, followed by the same measurement of the same domain. Phase-field simulation The total size of the simulation system was 750 × 750 × 1,300 nm 3 , which was discretized into a three-dimensional array of 150 × 150 × 260 cells. A cylindrical CFO particle with diameter d =500 nm and height h =300 nm in the middle of a BFO matrix ( Fig. 5a ) together with periodic boundaries was considered. Temporal evolution of the FE polarization in BFO and the magnetization in CFO was simulated by solving the time-dependent Ginzburg Landau equation [37] and the Landau–Lifshitz–Gilbert equation using a semi-implicit Fourier-spectral method [38] . The strain distribution in the nanocomposite system was obtained by solving the elastic equilibrium equation [39] with the stress-free strain ε 0 generated by electrostriction and magnetostriction calculated as and for the BFO and CFO phases, respectively; Q and λ were electrostrictive coefficient of BFO and saturation magnetostriction of CFO, respectively, which were taken as Q 11 =0.032 C −2 m 4 , Q 12 =−0.016 C −2 m 4 , Q 44 =0.020 C −2 m 4 , λ 100 =−590 p.p.m. and λ 111 =120 p.p.m. (ref. 35 ). How to cite this article: Li, Y. et al . Magnetoelectric quasi-(0-3) nanocomposite heterostructures. Nat. Commun. 6:6680 doi: 10.1038/ncomms7680 (2015).